Nanoscale memristive radiofrequency switches Radiofrequency switches are critical components in wireless communication systems and consumer electronics. Emerging devices include switches based on microelectromechanical systems and phase-change materials. However, these devices suffer from disadvantages such as large physical dimensions and high actuation voltages. Here we propose and demonstrate a nanoscale radiofrequency switch based on a memristive device. The device can be programmed with a voltage as low as 0.4 V and has an ON/OFF conductance ratio up to 10 12 with long state retention. We measure the radiofrequency performance of the switch up to 110 GHz and demonstrate low insertion loss (0.3 dB at 40 GHz), high isolation (30 dB at 40 GHz), an average cutoff frequency of 35 THz and competitive linearity and power-handling capability. Our results suggest that, in addition to their application in memory and computing, memristive devices are also a leading contender for radiofrequency switch applications. High-performance switches are critical components for the radiofrequency (RF) circuits that are widely used in wireless communications and consumer electronics [1] , [2] , [3] , [4] . Intense research in emerging switch technologies has focused on achieving levels of performance far beyond that available using CMOS (complementary metal oxide semiconductors) technology. Microelectromechanical system-based switches use a mechanical movement, usually activated by a voltage/current, to control an ohmic or capacitive contact [4] , [5] . Although superior to gallium arsenide and silicon-based switches in terms of energy consumption and transmission properties, microelectromechanical system switches suffer from issues such as speed, dielectric charging and contact interface degradation [4] , [5] . Other devices rely on recrystallization and amorphorization of a phase-change material (for example, germanium telluride) or the metal–insulator phase transition in strongly correlated materials (such as vanadium oxide, VO 2 ) to change the resistance state [6] , [7] , [8] , [9] . However, germanium telluride-based switches are constrained by a large switching energy and a limited resistance modulation ratio [6] , [7] , [8] . VO 2 has an insulator-to-metal transition temperature of 67 °C (refs 10 , 11 ) that limits the application of this device as a RF switch in a wider temperature range. Even worse is that the insulator phase transition in VO 2 is volatile, which means the device needs to be kept at above 67 °C to maintain a low-resistance state. Furthermore, most of the aforementioned emerging RF switches are of too large physical size to permit large-scale integration with nanometre CMOS RF circuits. Memristive devices are two-terminal resistance switches whose internal states are determined by the history of applied voltage and/or current [12] , [13] . Switching is typically related to the formation/rupture of one or more conductive filaments between two electrodes through either electrochemical reactions or the migration of mobile ions that modulate the interfacial properties [14] , [15] , [16] . These devices have demonstrated a number of attractive features, such as nonvolatility, low switching energy ( ∼ pJ; ref. 17 ), fast switching speed (<ns; ref. 18 ), high endurance (10 12 cycles) [19] , excellent scalability [20] , [21] , [22] and CMOS compatibility [25] . As such, memristive devices are promising candidates for universal memory [23] , [24] , reconfigurable bits [25] , nonvolatile logic [26] and unconventional computing [27] . Here we report a nanoscale RF switch based on a nonvolatile memristive device that consists of a pair of electrochemically asymmetric metal electrodes separated by a nanometre-scale air gap. Different from the aforementioned applications, RF circuits require a switch having low ON-state resistance ( R ON ) and low OFF-state capacitance ( C OFF ) to achieve a high cutoff frequency ( f c =1/2π R ON C OFF ) while maintaining sufficient linearity to be used in practical wide-band systems. In the design of our memristive RF switches, we realized that the R ON C OFF product is proportional to the product of the resistivity ( ρ ) of the conductive filament and the effective dielectric constant ( ɛ eff ) of the materials between the electrodes ( ρ·ɛ eff ). Consequently, we designed a device on thermally grown silicon oxide with two metal electrodes that are separated by an air gap. The active metal we used is silver (Ag), which has the lowest bulk resistivity ( ρ =1.59 × 10 −6 Ω cm) among all metals [2] , and the air gap on silicon oxide leads to a low effective dielectric constant ( ɛ eff ≈5.5) for the air–substrate interface in the active device region. The ability for the switch to function within an air gap, rather than a gap filled with the Ag-doped GeSe 2 film on which previous nanoionic switches have relied [28] , is enabled by the nanoscale feature size of the demonstrated device. Our memristive RF switch can be programmed with a voltage as low as 0.4 V and has an ON/OFF conductance ratio up to 10 12 . We also demonstrate low insertion loss (0.3 dB at 40 GHz), high isolation (30 dB at 40 GHz), a typical cutoff frequency of 35 THz and competitive linearity and power-handling capability. 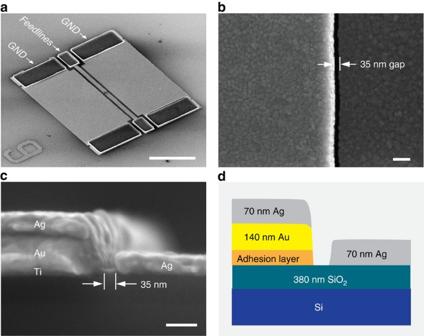Figure 1: The memristive RF switch is a planar device with two metal electrodes separated by a nanometre-scale gap. (a) A SEM image of the device with microscale thru lines and a nanoscale air gap. Scale bar, 100 μm. (b) Top-view SEM image of the 35-nm air gap (total length 8 μm). Scale bar, 200 nm. (c) Cross-sectional SEM image of the air gap between the two electrodes. Scale bar, 100 nm. (d) Schematic illustration of the geometry for the memristive RF device. The device is built on an intrinsic silicon wafer with 380-nm-thick thermally grown silicon dioxide. Device structure and programming Figure 1 shows the image and geometry of a typical memristive RF switch. It was fabricated on an intrinsic silicon wafer (resistivity>10,000 Ω cm) with a 380-nm-thick thermally grown silicon dioxide using photolithography, electron beam lithography (EBL) and tilted metal evaporation (see Methods, Supplementary Fig. 1 and Supplementary Note 1 for details). We used gold (Au) with a thin titanium (Ti) adhesion layer as one terminal and Ag as the other. The terminals were separated by a 35-nm-wide air gap. Figure 1: The memristive RF switch is a planar device with two metal electrodes separated by a nanometre-scale gap. ( a ) A SEM image of the device with microscale thru lines and a nanoscale air gap. Scale bar, 100 μm. ( b ) Top-view SEM image of the 35-nm air gap (total length 8 μm). Scale bar, 200 nm. ( c ) Cross-sectional SEM image of the air gap between the two electrodes. Scale bar, 100 nm. ( d ) Schematic illustration of the geometry for the memristive RF device. The device is built on an intrinsic silicon wafer with 380-nm-thick thermally grown silicon dioxide. Full size image Each terminal was connected to a much thicker (>1 μm) copper/aluminium (Cu/Al) pad to minimize the contact resistance with the measurement probes. Additional ground pads and metallization were fabricated at the same time to permit high-frequency characterization of the device within a well-defined coplanar waveguide (CPW) environment. The device exhibited nonvolatile bipolar resistance switching that crosses zero in the current–voltage curve, a signature of memristors ( Supplementary Fig. 2 and Supplementary Note 1 ). We used a voltage ramp (0 to 3 V or 0 to −0.4 V without return sweeps) to programme the device to the ON or OFF state. A current compliance ( I c ) was set to minimize the possible damage to the device without affecting the nonvolatility ( Fig. 2a ). By applying a maximum sweep voltage of 3 V to the Ag terminal relative to the Au/Ti terminal, a 110-nm-wide continuous Ag filament formed within the 35-nm gap ( Fig. 2b ). On the other hand, a −0.4-V bias ruptured the filament, programming the device in the OFF state ( Fig. 2c ). Both the high and low-resistance states (OFF/ON) after programming were nonvolatile, as confirmed by probing with lower voltages (±100 mV). In addition, the ON/OFF conductance ratio of the device was nearly 10 12 —7 orders of magnitude higher than that of a phase-change material switch [29] —indicating extremely low current flow in the OFF state. We further discovered that the geometry of the continuous silver filament was dependent on the programing process (see Supplementary Fig. 3 and Supplementary Note 2 ). Under otherwise identical conditions, a higher current led to a filament with larger diameter and hence lower resistance; however, this may also increase the energy required for programming. The filament formation initiates from the silver side, consistent with the electrochemical reaction mechanism [30] , [31] , [32] . However, previously reported devices with a similar structure but a larger gap size had considerably higher resistance because, rather than a continuous metal filament, isolated metal islands were formed between the electrodes [28] , [31] . We used a narrow gap and achieved a continuous filament with low resistance using low programming voltages. 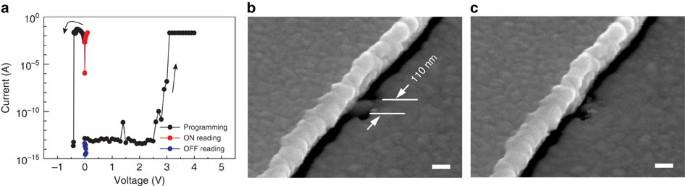Figure 2: The programming of the memristive RF switch is implemented with a dc voltage sweep and the ON and OFF states are achieved through the formation and rupture of a silver filament between the two electrodes. (a) Typical current–voltage curves for the SET and RESET processes for the device. A 3.0 V turned the device to the ON state, and a −0.4 V sweep turned the device OFF. The ON/OFF conductance ratio is nearly 1012. Note that the voltages are the applied value through the instrument. The red and blue dotted lines are the reading curves using −100 and 100 mV voltages after state changes, confirming the nonvolatility of the ON and OFF states. (b) SEM image of the device at the ON state. The metallic filament is made of silver and the diameter is 110 nm. (c) At the OFF state, the filament inbis ruptured, leaving a gap between the two metal electrodes. Scale bars, 100 nm. Figure 2: The programming of the memristive RF switch is implemented with a dc voltage sweep and the ON and OFF states are achieved through the formation and rupture of a silver filament between the two electrodes. ( a ) Typical current–voltage curves for the SET and RESET processes for the device. A 3.0 V turned the device to the ON state, and a −0.4 V sweep turned the device OFF. The ON/OFF conductance ratio is nearly 10 12 . Note that the voltages are the applied value through the instrument. The red and blue dotted lines are the reading curves using −100 and 100 mV voltages after state changes, confirming the nonvolatility of the ON and OFF states. ( b ) SEM image of the device at the ON state. The metallic filament is made of silver and the diameter is 110 nm. ( c ) At the OFF state, the filament in b is ruptured, leaving a gap between the two metal electrodes. Scale bars, 100 nm. Full size image Device-retention properties We did not observe device failure from OFF to ON state up to 200 °C. To evaluate the ON state retention of the memristive RF switches, we measured the failure time of ON-state devices at different temperatures. The device under test was programmed to low resistance at room temperature and then mounted on a closed loop thermal chuck with an accuracy of ±0.5 °C. The resistance of each device was measured using a semiconductor parameter analyser once every 5 minutes until the current dropped dramatically. 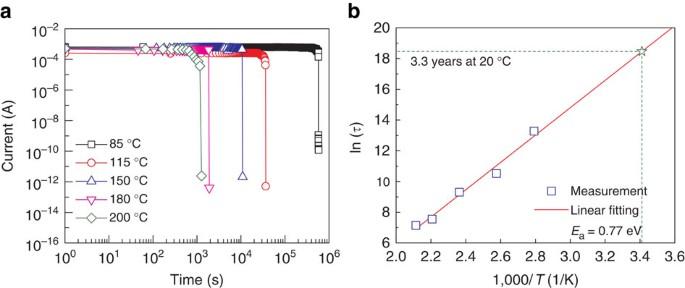Figure 3: Retention properties of the memristive RF switch. (a) Retention measurement of ON states at 85, 115, 150, 180 and 200 °C. (b) Temperature dependence of the retention failure time (τ) follows the Arrhenius relation. Retention at 20 °C extrapolated from the linear fitting of measurement results was∼3.3 years (marked by a star). The activation energyEais calculated to be 0.77 eV. Figure 3a shows the measured retention time for our devices at 85, 115, 150, 180 and 200 °C, which ranged from 5 × 10 5 to ∼ 10 3 s. We found that the retention time ( τ ) followed an Arrhenius relation [33] with respect to temperature ( T ), 1/ τ ∝ exp(− E a / kT ), where E a is the activation energy for the Ag diffusion and k the Boltzmann constant. By extending the fitted results to room temperature (20 °C), the expected retention time of our device was beyond 3.3 years ( Fig. 3b ). The long retention time is likely due to the very low mobility of Ag atoms on the surface and inside of silicon oxide (4.5 × 10 −13 cm 2 s −1 ) at room temperature [34] . It should be pointed out that the retention measurement in this study was conducted in air without passivation or other hermetic protection. The ‘failed’ devices tested at or below 150 °C could still be SET to the low-resistance state using a voltage sweep as described in Fig. 2a , indicating that the switching was nondestructive. The retention time could be further improved by introducing a hermetic seal around the device. Figure 3: Retention properties of the memristive RF switch. ( a ) Retention measurement of ON states at 85, 115, 150, 180 and 200 °C. ( b ) Temperature dependence of the retention failure time ( τ ) follows the Arrhenius relation. Retention at 20 °C extrapolated from the linear fitting of measurement results was ∼ 3.3 years (marked by a star). The activation energy E a is calculated to be 0.77 eV. Full size image The E a extracted from Fig. 3b is 0.77 eV, which lies between the value reported for Ag diffusion on SiO 2 surface (0.30–0.44 eV; refs 35 , 36 , 37 ) and that for Ag diffusion inside SiO 2 ( ∼ 1.24 eV; ref. 34 ). The intermediate activation energy suggests that part of the conductive Ag filament was embedded in the SiO 2 substrate during the diffusion process. This is consistent with previous observations that Ag diffusion occurs both on the SiO 2 surface and inside of the SiO 2 simultaneously [38] . Temperature and humidity effects on programming voltages The switching behaviour is dependent on the ambient temperature. As shown in Fig. 4a , the SET voltage decreased with higher temperatures, while the RESET voltage was insensitive to the ambient temperature. This implies that a higher temperature favours the formation of an Ag filament during the SET process [39] . The RESET process is dictated by Joule heating and the ambient temperature does not significantly affect the fracturing of the filament. The temperature dependency suggests that a lower programming voltage is needed when the device is used for RF circuits that operate at 85 °C or above. Furthermore, the programming voltage is also affected by the environment humidity ( H r ): the SET voltage decreased with higher H r while the RESET voltage remained almost unchanged ( Fig. 4b ). The strong correlation between the SET voltage and the humidity could be explained both by the critical role of moisture in the Ag ionization at the anode and by the migration of Ag ions during the SET process. At higher humidity levels, more water molecules are absorbed on the SiO 2 surface. A dense hydrogen-bond network is hence formed that provides necessary counter charges for Ag ionization [40] and lowers the activation energy for Ag ion migration, leading to a smaller SET voltage. On the other hand, the RESET process of our device originates from filament fracture due to strong Joule heating and is thus less influenced by moisture. It is worthwhile to point out that the ambient humidity also affects the device endurance (see Supplementary Fig. 4 and Supplementary Note 3 ). 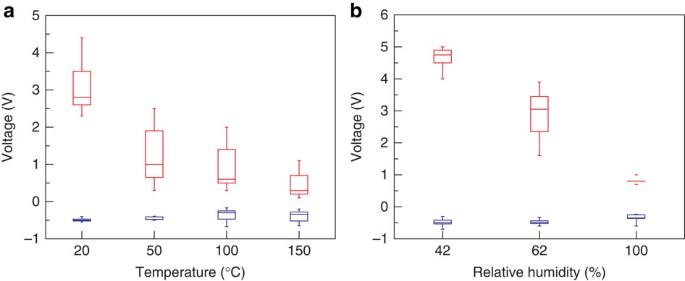Figure 4: Temperature and humidity dependence of the programming voltages. The SET voltage (red) decreases with the temperature (a) and relative humidity (b), while the RESET voltage (blue) does not change noticeably with these two factors. The temperature dependency was studied under a constant humidity of 50%. For the study of humidity dependence, the ambient relative humidity (Hr) was 42% (clean room ambient), 62% (water vapour) and 100% (DI water immersion), respectively, while the temperature was fixed at 20 °C. Boxplot explanation: upper and lower box hinges 75 and 25 percentiles; the upper and lower whiskers indicate 99 and 1 percentiles, respectively; the horizontal line within box represents the median; the small box shows the average value. Figure 4: Temperature and humidity dependence of the programming voltages. The SET voltage (red) decreases with the temperature ( a ) and relative humidity ( b ), while the RESET voltage (blue) does not change noticeably with these two factors. The temperature dependency was studied under a constant humidity of 50%. For the study of humidity dependence, the ambient relative humidity ( H r) was 42% (clean room ambient), 62% (water vapour) and 100% (DI water immersion), respectively, while the temperature was fixed at 20 °C. Boxplot explanation: upper and lower box hinges 75 and 25 percentiles; the upper and lower whiskers indicate 99 and 1 percentiles, respectively; the horizontal line within box represents the median; the small box shows the average value. Full size image RF performance measurement and modelling We measured the RF performance of our devices up to 110 GHz using a vector network analyser (VNA). A multiline thru-reflect-line (TRL) calibration using a set of on-wafer standards ( Supplementary Fig. 5 and Supplementary Note 4 ) was used to place the measurement reference plane 5 μm away from the edge of the intrinsic device [41] , [42] . The transmission spectra of 33 devices were obtained. In a 50-Ω environment, the average OFF-state isolation and ON-state insertion loss at 40 GHz were 30 and 0.33 dB, respectively (example curves and statistical metrics appear in Fig. 5 ). At higher frequencies, the OFF-state measurement was limited by weak coupling to undesired modes supported by the intrinsic silicon substrate. This coupling could be eliminated if the switch were integrated in a thin-film grounded CPW structure ( Supplementary Fig. 6 and Supplementary Note 5 ). 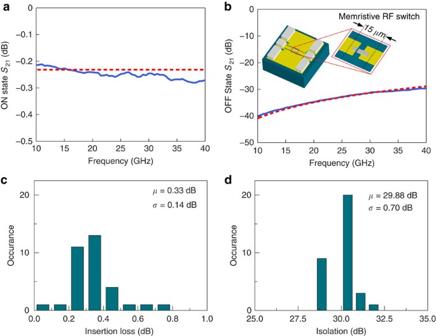Figure 5: Transmission characterization of the memristive RF switch. (a) Typical transmission spectrum of a device at the ON state (solid blue line) with fittings from the equivalent circuit model (dashed red line). The insertion loss at 40 GHz for this device is lower than 0.3 dB. (b) Transmittance spectrum of the device at the OFF state (solid blue line) with fittings from equivalent circuit model (dashed red line). The isolation at 40 GHz is∼30 dB. The inset shows the device structure and the reference planes (dotted lines) used for de-embedding. For both ON and OFF state measurements, padframe and feedline parasitics have been de-embedded to expose the intrinsic switch performance. (c,d) The statistics for the insertion loss and isolation at 40 GHz for the 33 devices we measured.μandσare the mean value and s.d., respectively. Figure 5: Transmission characterization of the memristive RF switch. ( a ) Typical transmission spectrum of a device at the ON state (solid blue line) with fittings from the equivalent circuit model (dashed red line). The insertion loss at 40 GHz for this device is lower than 0.3 dB. ( b ) Transmittance spectrum of the device at the OFF state (solid blue line) with fittings from equivalent circuit model (dashed red line). The isolation at 40 GHz is ∼ 30 dB. The inset shows the device structure and the reference planes (dotted lines) used for de-embedding. For both ON and OFF state measurements, padframe and feedline parasitics have been de-embedded to expose the intrinsic switch performance. ( c , d ) The statistics for the insertion loss and isolation at 40 GHz for the 33 devices we measured. μ and σ are the mean value and s.d., respectively. Full size image We analysed the small-signal performance of the nanoscale memristive switch using a simple physics-based lumped-element equivalent circuit model shown in Fig. 6a . This equivalent circuit model was extracted for each device and used to compute the switch cutoff frequencies. Statistics for the R ON , C OFF and f c are provided in Fig. 6b–d . Among the 33 measured devices, the R ON of the intrinsic switch has a mean value of 3.6 Ω and varies from 2.1 to 6.9 Ω. According to electromagnetic simulations, the extracted range of ON-state resistance corresponds to nanofilaments with cross-sections varying from ∼ 5 × 10 −12 to 80 × 10 −12 cm 2 . The C OFF of ∼ 1.4 fF is predominantly associated with the capacitance of the 35-nm gap, which depends on the effective dielectric constant of the substrate–air interface. This number is consistent with both electromagnetic simulations and simple hand calculations (see Discussion and Supplementary Note 6 ). The average value of f c is 35 THz and can be further enhanced if an identical device were fabricated at the top of a typical CMOS metal stack that has a much thicker SiO 2 layer. Further enhancement of the small-signal performance could also be achieved by controlling the filament geometry to reduce R ON . 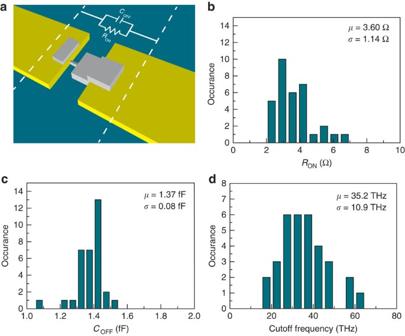Figure 6: Device modelling and performance statistics for 33 measured devices. (a) Schematic illustration of the device in the ON state with equivalent circuit model. The device is modelled as a resistor (RON) connected in parallel with a capacitor (COFF) between the silver and gold electrodes. (b–d) Statistics for the extracted ON-state resistance (RON) (b), OFF-state capacitance (COFF) (c) and cutoff frequency (fc) (d). The average values ofRON,COFFandfcare 3.6 Ω, 1.37 fF and 35.2 THz, respectively. Figure 6: Device modelling and performance statistics for 33 measured devices. ( a ) Schematic illustration of the device in the ON state with equivalent circuit model. The device is modelled as a resistor ( R ON ) connected in parallel with a capacitor ( C OFF ) between the silver and gold electrodes. ( b–d ) Statistics for the extracted ON-state resistance ( R ON ) ( b ), OFF-state capacitance ( C OFF ) ( c ) and cutoff frequency ( f c ) ( d ). The average values of R ON , C OFF and f c are 3.6 Ω, 1.37 fF and 35.2 THz, respectively. Full size image We also evaluated the linear performance of the switches using a VNA capable of standard two-tone distortion measurements. The third-order intermodulation intercept in the ON- and OFF-states was evaluated using measurements of series and shunt switches to capture a realistic operating environment corresponding to a single-pole double throw switch. In both cases, we found that the third-order intermodulation intercept was beyond the measurement limit of +45 dBm ( Supplementary Figs 7 and 8 and Supplementary Note 7 ). Self-switching evaluation RF-induced resistance switching is another potential concern with a memristive switch due to the sub-1 V actuation voltage of these devices. We evaluated the feasibility for self-switching under RF power by exciting both ON- and OFF-state devices and capturing scanning electron microscopy (SEM) photos as we gradually increased the RF power ( Fig. 7a,b ). A frequency of 5 GHz was selected for these measurements. We observed no evidence of self-switching in measurements of the OFF-state device up to the maximum available generator power of +21 dBm. However, when measuring the ON-state device, we observed self-switching at a power level above +17 dBm. We also investigated the dependence of self-switching on the frequency of excitation by measuring a variety of devices exited with RF energy at 10, 100 and 1,000 MHz. In all cases, we found that OFF state devices were not susceptible to self-switching. Moreover, we observed little correlation between ON-state power-handling capability and RF excitation frequency. Instead, we observed a strong dependence between the ON-state resistance and the power at which the device self-actuated ( Fig. 7c ). The inverse relationship between power handling and ON-state resistance is consistent with a Joule heating-based reset mechanism and indicates that power handling can be improved by engineering nanofilaments with reduced ON-state resistance (see Supplementary Note 6 for further analysis). 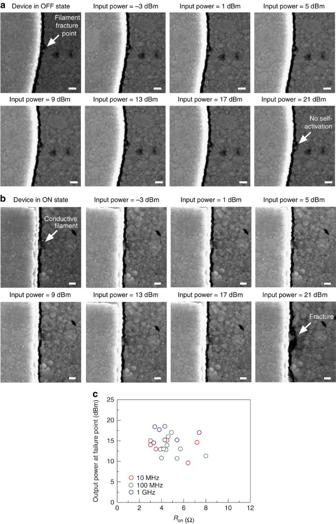Figure 7: Power-handling capability of the memristive RF switch. (a) SEM images of devices at the OFF state after tested under different RF input powers at 5 GHz. No self-activation was observed during the measurement. (b) Device at the ON state starts self-switching at 17 dBm. The diameter of the filament was 95 nm. Scale bars, 100 nm. (c) Output power at which the self-switching occurs for on devices versus on resistance for 10 MHz, 100 MHz and 1 GHz. Increasing the filament diameter will improve the RF power-handling capability for devices in the ON state. Figure 7: Power-handling capability of the memristive RF switch. ( a ) SEM images of devices at the OFF state after tested under different RF input powers at 5 GHz. No self-activation was observed during the measurement. ( b ) Device at the ON state starts self-switching at 17 dBm. The diameter of the filament was 95 nm. Scale bars, 100 nm. ( c ) Output power at which the self-switching occurs for on devices versus on resistance for 10 MHz, 100 MHz and 1 GHz. Increasing the filament diameter will improve the RF power-handling capability for devices in the ON state. Full size image To further understand the potential of the memristive devices as RF switches, we verified the ON- and OFF-state parameters using a full-wave electromagnetic simulation carried out in ANSYS High-Frequency Structural Simulator (ANSYS Inc., Canonsburg, Pennsylvania). A frequency range of 1–200 GHz was selected and the substrate was made sufficiently small to avoid substrate-moding effects. A wave-port de-embedding was employed to set the reference plane of the simulation to that of the experimental measurement. The CPW feedline cross-section and silver electrodes were made identical to the fabricated structures and a 35-nm gap was selected for the active memristor region. For ON-state simulations, a small rectangular silver filament was used to short the gap. The conductivity of the silver was reduced by a factor of three from its bulk value to account for nanoscale effects [43] . The thickness and width of the filament were varied to study the impact of the filament dimension on the ON-state resistance. The predicted OFF-state transmission appears in Fig. 8a . At 40 GHz, the predicted isolation is 31 dB, which is within 1 dB of the measured value (30 dB) as shown in Fig. 5 . Moreover, the predicted isolation remains better than 17 dB to 200 GHz. The OFF-state capacitance was calculated as C OFF =–imag{1/ Y 12 }/ ω . The result is plotted in Fig. 8b . Over a broad range of frequencies, the predicted capacitance is 1.17 fF, which is consistent with both hand calculations and measurement. Moreover, the frequency independence of the extracted capacitance validates our use of the simple lumped element equivalent circuit. 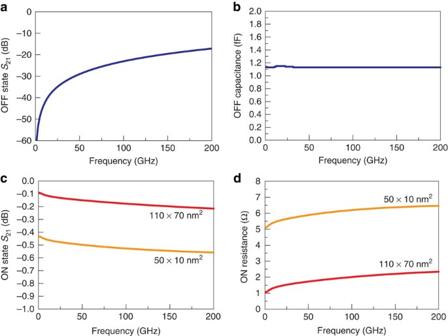Figure 8: Electromagnetic simulation results using High-Frequency Structural Simulator (HFSS). (a) OFF-state transmission; (b) OFF-state capacitance; (c) ON-state transmission; and (d) ON-state resistance for two filament cross-sections. Figure 8: Electromagnetic simulation results using High-Frequency Structural Simulator (HFSS). ( a ) OFF-state transmission; ( b ) OFF-state capacitance; ( c ) ON-state transmission; and ( d ) ON-state resistance for two filament cross-sections. Full size image The simulated transmission of the ON-state device is shown in Fig. 8c for filaments with cross-sections of 110 nm × 70 nm and 50 nm × 10 nm. The average experimentally obtained insertion loss value (0.33 dB) corresponds to a nanofilament of cross-section 8 × 10 −12 cm 2 , which is significantly smaller than expected based on SEM imaging. This indicates that a significant component of the RF resistance may be related to contact resistance. The corresponding ON-state resistance is plotted versus frequency in Fig. 8d . The memristive RF switch requires no power to maintain the ON or OFF state, potentially leading to power efficiency advantages. The low programming voltage enables monolithic integration of memristive RF switches with low-power CMOS circuits to expand the functionality. The device fabrication process for our memristive RF switches is also simpler as compared with other devices. Further scaling of the device, such as shrinking the gap size, will lead to optimized switching behaviour such as longer endurance and lower power consumption [44] , [45] with no degradation to the RF performance, provided the ON-state resistance is dominated by the filament and not other effects. It is necessary to engineer the location and geometry of the metallic filaments for even lower ON-state resistance, to enhance the device endurance, and to reduce the energy required for each switching event. Nonetheless, we believe that memristive RF switches will become one of the leading contenders in RF circuits for communication and consumer electronics. Device geometry and fabrication The memristive RF switches were built on an intrinsic silicon wafer (resistivity>10,000 Ω cm) with a 380-nm-thick thermally grown oxide. The fabrication procedure involved three major steps that defined the microscale contact pads, the CPW structure and the nanoscale gap. The microscale features were patterned by photolithography using 365-nm wavelength ultraviolet radiation, and the nanogap was defined using EBL. The padframe and feedline structures consisted of a 10-nm-thick Ti adhesion layer and a 140-nm-thick gold layer, both deposited in an electron beam evaporator. The distance between the central electrodes was 5 μm. The contact pads were made of 1-μm-thick Cu and 500-nm-thick Al that were deposited by RF magnetron sputtering. Before fabricating the nanometre-scale gap, a rectangular window of 30 μm by 8 μm was opened by EBL in the centre area of the electrodes. The nanogap was created by evaporating 70-nm-thick Ag with a tilted angle. For the 35-nm gap, the evaporation angle was 65° relative to the wafer surface. See Supplementary Note 1 for the detailed fabrication procedure and schematics. DC programming The devices were programmed to the ON- or OFF-state with quasi-DC voltage sweeps using a Keithley 4200SC semiconductor parameter analyser. A current compliance was set to protect the device, and to control the size and morphology of the metallic filament. During the programming, the inert metal electrode was grounded and the silver electrode was biased. A positive voltage will SET the device to a low resistance by bridging the nanogap, while a negative voltage ruptures the filament and RESETs the device to the high-resistance state. RF measurements Small-signal measurements were carried out ON-wafer using an Agilent N5247A VNA with a pair of N5260 frequency extender modules, permitting measurements to be carried out from 0.01 to 110 GHz. To minimize substrate-moding when measuring the OFF-state-scattering parameters, the switches were first singulated to a size of ∼ 1 mm × 1 mm × 0.55 mm (length × width × height) and then mounted using photo-resist on a rigid absorber composed of carbon-loaded epoxy. For small-signal measurements, the RF power was set to a nominal level of −5 dBm. A multiline TRL calibration was carried out from 10 to 110 GHz using a set of standards fabricated on an identical substrate as the memristive switches (further details are provided in the Supplementary Note 4 ). The multiline TRL calibration [41] , [42] placed the measurement reference plane 5 μm from the edge of the intrinsic device. No additional de-embedding was employed. A second calibration using the LRM+ algorithm carried out on a Cascade 104-783 calibration substrate was employed to measure the devices, referenced at the plane of the bondpads so that a comparison of the ON-state device to a thru line could be made ( Supplementary Fig. 9 and Supplementary Note 8 ). All calibrations were performed using Cascade WinCal software (Cascade Microtech Inc., Beaverton, Oregon), before device measurement, allowing for data at the two reference planes to be acquired simultaneously. Scattering parameters were collected for each device in both the ON- and OFF-states, and parameter extraction was carried out to determine the ON- and OFF-state equivalent circuit models. Two-tone linearity measurements were carried out at 5 GHz with a 1-MHz-tone spacing and a swept power level ranging from −30 to +7 dBm. Power handling was evaluated in the ON- and OFF-states by driving the memristor with a laboratory CW source (Agilent PSG8257D) and measuring the output power using a spectrum analyser (Agilent N9010A). The power was swept from −20 to +21 dBm, with steps of 1 dBm for three different frequencies including 10 MHz, 100 MHz and 1 GHz. All cable losses were determined and de-embedded. The detailed evolution of one ON-state and one OFF-state device was studied by incrementally capturing SEM images as the devices were gradually exposed to higher RF power levels. For this experiment the RF power swept from −3 to 21 dBm with steps of 4 dBm and the frequency was set to 5 GHz. SEM photos were obtained at each step. How to cite this article: Pi, S. et al . Nanoscale memristive radiofrequency switches. Nat. Commun. 6:7519 doi: 10.1038/ncomms8519 (2015).